Alternative splicing regulates vesicular trafficking genes in cardiomyocytes during postnatal heart development During postnatal development the heart undergoes a rapid and dramatic transition to adult function through transcriptional and post-transcriptional mechanisms, including alternative splicing (AS). Here we perform deep RNA-sequencing on RNA from cardiomyocytes and cardiac fibroblasts to conduct a high-resolution analysis of transcriptome changes during postnatal mouse heart development. We reveal extensive changes in gene expression and AS that occur primarily between postnatal days 1 and 28. Cardiomyocytes and cardiac fibroblasts show reciprocal regulation of gene expression reflecting differences in proliferative capacity, cell adhesion functions and mitochondrial metabolism. We further demonstrate that AS plays a role in vesicular trafficking and membrane organization. These AS transitions are enriched among targets of two RNA-binding proteins, Celf1 and Mbnl1, which undergo developmentally regulated changes in expression. Vesicular trafficking genes affected by AS during normal development (when Celf1 is downregulated) show a reversion to neonatal splicing patterns after Celf1 re-expression in adults. Short-term Celf1 induction in adult animals results in disrupted transverse tubule organization and calcium handling. These results identify potential roles for AS in multiple aspects of postnatal heart maturation, including vesicular trafficking and intracellular membrane dynamics. The heart is the first organ to form and function during vertebrate embryogenesis [1] . The first 4 postnatal weeks involve a period of extensive physiological remodelling with dynamic changes as the fetal heart adapts to birth and converts to adult function. This transition occurs through transcriptional and post-transcriptional mechanisms, including coordinated networks of alternative splicing (AS) [1] , [2] , [3] , [4] . Human and rat hearts are composed of 66% cardiac fibroblasts (CF), 30% cardiomyocytes (CM) and 4% endothelial and vascular smooth muscle cells [5] , [6] , [7] . Studies differ regarding adult mouse heart composition. While Soonpaa et al. [8] reported that CF account for 86% of cells, a recent analysis demonstrated a composition of 26% CF, 56% CM and 18% non-CM and non-CF [9] . However, CM comprise ~75% of the tissue volume in mammals [7] . CM generate the contraction force and CF form the mechanical scaffold required for effective pumping [10] . CM and CF communicate through multiple signalling mechanisms and through extracellular matrix (ECM) [11] . Other CF functions include response to cardiac injury [12] and electrical isolation of different regions of the cardiac conduction system [13] . By postnatal day 7 (PN7), CM lose proliferative capacity and heart size increases due to CM hypertrophy [14] , [15] . Limited microarray analysis of messenger RNA expression in freshly isolated CM and CF showed that while certain genes are highly expressed in CM, many growth factors, cytokines and ECM genes are more highly expressed in CF [16] . Overall, the published data address a limited number of gene expression changes in CM and CF during development and, notably, do not provide AS information. High-throughput studies of AS and gene expression regulation have primarily focused on differences between tissues, normal versus pathological conditions or cultured cells. A small set of reports have addressed AS and gene expression changes during normal physiological transitions [17] , [18] , [19] , [20] , [21] . Development provides an outstanding opportunity to identify coordinated AS regulation critical for physiological transitions from embryonic to adult functions. Previously, we showed that genes that undergo AS regulation during heart development produce transitions from embryonic to adult protein isoforms largely without changes in overall transcript levels, presenting a new paradigm for understanding developmentally regulated gene expression in the heart [3] . Nearly half of the AS transitions identified in mouse are conserved during post-hatch chicken heart development, suggesting highly conserved functions for splicing-mediated isoform transitions [3] . In the present study, we analysed AS and gene expression transitions regulated during postnatal mouse heart development using mRNA deep sequencing (RNA-seq) [22] . To gain insight into the diversity of cell type-specific transitions, we performed RNA-seq using freshly isolated CF and CM from a developmental time course. The results reveal that most gene expression and AS changes occur within the first 4 weeks after birth, and that CM and CF exhibit reciprocal transitions in expression of specific functional categories (proliferation, cell adhesion, cytokines-chemotaxis, metabolism and transcription regulation). Interestingly, we found that genes involved in vesicular trafficking and membrane organization are regulated by AS during postnatal CM development. These AS changes are enriched as targets of the CUGBP, ELAV-like family (Celf) and Muscleblind-like (Mbnl) RNA-binding protein families, both of which are involved in AS and are regulated during postnatal heart development [3] , [23] , [24] . In the heart, vesicular trafficking-related AS transitions probably impact ligand/growth factor uptake, ion channels dynamics and/or postnatal formation of the sarcoplasmic reticulum (SR) and transverse tubules (T-tubules), crucial processes for excitation-contraction coupling (ECC) that are established by PN30 (ref. 25 ). We show that re-expression of CELF1 in adults specifically in CM results in altered T-tubule structure and misregulated calcium handling consistent with alterations associated with re-expression of fetal splicing patterns. Extensive transcriptome changes during postnatal development RNA-seq was performed using RNA from mouse ventricles isolated at five time points: E17, PN1, PN10, PN28 and adult (PN90). Complementary DNA libraries were prepared after ribosomal RNA (rRNA) depletion for 100 bp paired-end reads using the Illumina HiSeq2000. 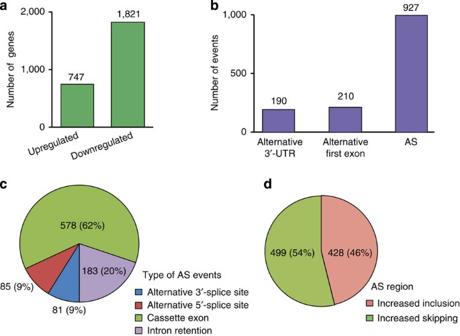Figure 1: Extensive gene expression and RNA processing changes occur during heart development. (a,b) Differentially expressed genes (a) and alternative RNA processing between E17-adult (b). (c) AS events categorized by pattern. (d) Proportion of skipping/inclusion of the AS regions. AS, alternative splicing. We obtained >150 million read pairs per sample, >80% of which mapped the mouse genome ( Supplementary Table 1 ). We identified 2,568 differentially expressed genes (≥2.0-fold, false discovery rate: 0.01, see Methods) between E17-adult: 747 were upregulated and 1,821 were downregulated ( Fig. 1a ). Analysis of mRNA isoforms whose percent spliced in (PSI) [26] values changed ≥20% (ΔPSI≥20%) between E17-adult identified 927 AS events, 190 alternative 3′-untranslated regions (UTRs) and 210 alternative first exons ( Fig. 1b ). Postnatal AS transitions were predominantly cassette exons (62%), while alternative 3′- and 5′-splice sites each represented 9%. We observed a relatively high proportion of transitions (20%) involving intron retention with roughly equal proportions of events exhibiting increased inclusion or exclusion of the variable regions during development ( Fig. 1c,d ). Figure 1: Extensive gene expression and RNA processing changes occur during heart development. ( a , b ) Differentially expressed genes ( a ) and alternative RNA processing between E17-adult ( b ). ( c ) AS events categorized by pattern. ( d ) Proportion of skipping/inclusion of the AS regions. AS, alternative splicing. Full size image Extensive remodelling within the first 4 weeks after birth Gene ontology (GO) analysis of downregulated genes between E17-adult in ventricles showed a clear enrichment ( P <1E−10, Fisher exact test) in categories related with cell cycle and DNA replication ( Fig. 2a , left). As ~75% of ventricular RNA originates from CM [7] , this is consistent with the loss of CM proliferative activity by PN7 (refs 14 , 15 ). Upregulated genes between E17-adult showed enrichment in categories related to mitochondria, fatty-acid metabolism and oxidation-reduction processes ( Fig. 2a , right) consistent with increased mitochondrial number and the metabolic switch from carbohydrates to fatty acids, a hallmark of the fetal to adult CM metabolic transition [27] , [28] . 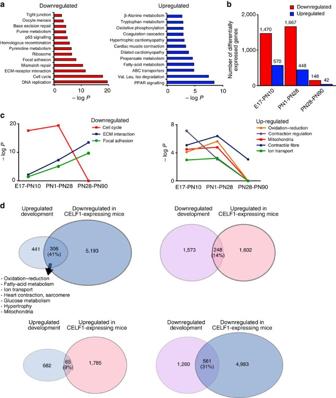Figure 2: Gene expression regulation occurs primarily before PN28. (a) GO analysis (Kyoto Encyclopedia of Genes and Genomes (KEGG) pathways) of down- and upregulated genes between E17-adult (ventricles). (b) Differentially expressed genes between E17–PN10, PN1–PN28 and PN28–PN90 (ventricles). (c) Significance of KEGG pathways (−logP) were plotted against time windows for specific categories. (d) Venn diagrams with developmentally regulated genes and those regulated after CELF1 re-expression on adult mice (RNA-seq data). GO analysis of the intersected genes (summary). ECM, extracellular matrix;P, Fisher exactPvalue. Figure 2: Gene expression regulation occurs primarily before PN28. ( a ) GO analysis (Kyoto Encyclopedia of Genes and Genomes (KEGG) pathways) of down- and upregulated genes between E17-adult (ventricles). ( b ) Differentially expressed genes between E17–PN10, PN1–PN28 and PN28–PN90 (ventricles). ( c ) Significance of KEGG pathways (−log P ) were plotted against time windows for specific categories. ( d ) Venn diagrams with developmentally regulated genes and those regulated after CELF1 re-expression on adult mice (RNA-seq data). GO analysis of the intersected genes (summary). ECM, extracellular matrix; P , Fisher exact P value. Full size image Analysis of three time windows (E17–PN10, PN1–PN28 and PN28–PN90) revealed that the majority of gene expression transitions occurred before PN28 ( Fig. 2b ). Enrichment analysis in each period showed that downregulation of cell cycle-related genes occurred before PN28 (−log P dropped off after PN28; Fig. 2c , left) in agreement with the loss of CM proliferative capacity early after birth. Similarly, upregulated genes related to mitochondria, fatty-acid metabolism and oxidation-reduction were more enriched before PN28 ( Fig. 2c , right). In contrast, categories such as focal adhesion and ECM-receptor interaction were more enriched after PN28 in downregulated genes (−log P increased after PN28; Fig. 2c , left). Detailed analysis of individual cell cycle and ECM genes confirmed temporal differences in downregulation. The majority of ECM-related genes maintained high mRNA levels within the first 10 days after birth, dropped off at PN28 and decreased further in adults, while 81% of cell cycle genes were strongly downregulated before PN10 ( Supplementary Fig. 1a,b ). The 3′-UTRs of downregulated ECM- and cell cycle-related genes were computationally analysed for putative microRNA (miRNA) miR-15 and miR-29 seed sequences. While 41% of the downregulated ECM genes were predicted to be miR-29 targets, 33% of the downregulated cell cycle genes were predicted to be miR-15 targets. These results suggest that a possible mechanism for the distinct patterns of cell cycle and ECM downregulation could involve miRNAs since these transcripts are well-established targets of developmentally upregulated miRNAs such as miR-15 and miR-29 families [29] , [30] , [31] , [32] . Celf1 loss correlates with increased expression of gene sets To investigate a mechanism of upregulation during postnatal development, we explored a potential role for Celf1, a RNA-binding protein downregulated 10-fold during the first 2 weeks after birth [3] . Celf1 binds to GU-rich motifs within introns regulating AS [3] , [33] and within 3'-UTRs promoting mRNA decay [34] , [35] . To identify genes that are responsive to Celf1 expression during postnatal development, we used previously described tetracycline-inducible transgenic mice ( TRECUGBP1/MHC ) to induce human CELF1 expression in CM [33] . RNA-seq was performed using ventricles of adult TRECUGBP1/MHC and control (MHC; myosin heavy chain) littermates after 12, 24, 72 h or 7 days of induction. A high fraction (41%) of the developmentally upregulated genes was downregulated within 72 h of exogenous CELF1 re-expression in adults ( Fig. 2d , left). While a large number of genes are downregulated after CELF1 induction (5,499), the majority (93%) of them shows a relatively small change (≤2.0-fold, after 72 h). In contrast, a high fraction (78%) of the 306 overlapping genes (upregulated during development and downregulated by CELF1 expression) shows a fold change ≥2.5, suggestive of a physiological response. Developmentally upregulated genes responsive to CELF1 (306 genes) were enriched in oxidation-reduction pathways, fatty-acid metabolism, mitochondria and sarcomere related categories. By contrast, only 14% of developmentally downregulated genes were affected by CELF1 re-expression ( Fig. 2d ), suggesting that a percentage of the developmentally upregulated mRNAs are destabilized by CELF1. A high proportion of the developmentally downregulated genes overlapped with the downregulated genes after CELF1 induction ( Fig. 2d , bottom right). However, CELF1-downregulated genes show only 31% overlap with developmental downregulated genes compared with 41% overlap with developmentally upregulated genes suggesting that Celf1 postnatal downregulation stabilizes a large subset of mRNAs. It is also likely that there are secondary consequences to CELF1 re-expression (such as effects on transcription factor expression) resulting in both positive and negative effects on mRNA levels. To further investigate the potential CELF1 role in regulating mRNA stability during postnatal development, we analysed the 3′-UTRs of 58 genes in the oxidation-reduction and mitochondria categories for CELF1-binding motifs ( Supplementary Fig. 1c,d ). The GU-rich motif shown in Supplementary Fig. 1c was significantly enriched ( E =2.5E−05) and present in 24% of the analysed 3′-UTRs. A similar GU-rich motif was found by CLIPZ with a high level of enrichment ( Supplementary Fig. 1d ). CLIPZ and MEME (Multiple Em Motif Elicitation) analysis also identified enrichment of polyA and GGA motifs ( Supplementary Fig. 1c,d ). These results suggest that postnatal Celf1 downregulation promotes upregulation of genes within specific functional pathways through mRNA stabilization. Transcriptome changes in CM and CF during development To identify cell type-specific transitions, we isolated CM and CF from ventricles of PN1–3, PN28–30 and adult (PN60–67) animals. RNA was extracted from CM and CF cell populations within 3 h of animal euthanasia to reduce post-mortem and cell manipulation effects. CF from all developmental stages and neonatal CM were isolated by an enzymatic digestion/pre-plating method. Adult and PN30 CM were isolated by Langendorff perfusion (see Methods). Morphology, binucleation (CM) and positive immunostaining for alpha-actinin (CM) and vimentin (CF) from adult animals were confirmed by confocal and differential interference contrast microscopy ( Fig. 3a ). Reverse transcription–PCR (RT–PCR) analysis of cell-specific markers in adult CM and CF demonstrated a high degree of purity ( Fig. 3b ). Analysis of cell-specific markers in RNA-seq data confirmed these results demonstrating similar purity levels for early and late postnatal stages (see below). 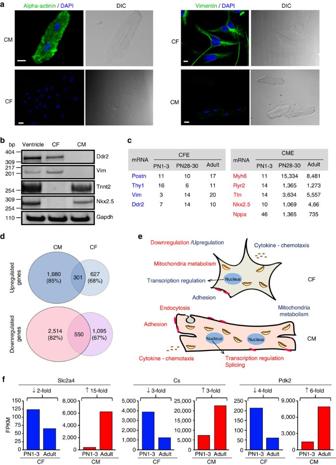Figure 3: Reciprocal gene expression transitions between CM and CF. (a) Isolated adult ventricular CM and CF stained with anti-vimentin or anti-alpha-actinin. Scale bar, 10 μm. (b) RT–PCR assays of CF (Vim, Ddr2) and CM (Tnnt2, Nkx2.5) markers on RNA from adult ventricles, CM and CF. Experiments were repeated with at least three independent samples. (c) CF enrichment (CFE) for CF-enriched transcripts (blue) and CM enrichment (CME) for CM-enriched transcripts (red) calculated from RNA-seq data. (d) Postnatal gene expression transitions in CM and CF (PN1–3 versus adult) by RNA-seq. (e) GO analysis of down- and upregulated genes in CM and CF (Supplementary Table 2). (f) Postnatal expression of three metabolic genes (RNA-seq data) showing reciprocal CM–CF regulation. bp, base pairs; DIC, differential interference contrast microscopy; FPKM, fragments per kilobase per million mapped. Figure 3: Reciprocal gene expression transitions between CM and CF. ( a ) Isolated adult ventricular CM and CF stained with anti-vimentin or anti-alpha-actinin. Scale bar, 10 μm. ( b ) RT–PCR assays of CF (Vim, Ddr2) and CM (Tnnt2, Nkx2.5) markers on RNA from adult ventricles, CM and CF. Experiments were repeated with at least three independent samples. ( c ) CF enrichment (CFE) for CF-enriched transcripts (blue) and CM enrichment (CME) for CM-enriched transcripts (red) calculated from RNA-seq data. ( d ) Postnatal gene expression transitions in CM and CF (PN1–3 versus adult) by RNA-seq. ( e ) GO analysis of down- and upregulated genes in CM and CF ( Supplementary Table 2 ). ( f ) Postnatal expression of three metabolic genes (RNA-seq data) showing reciprocal CM–CF regulation. bp, base pairs; DIC, differential interference contrast microscopy; FPKM, fragments per kilobase per million mapped. Full size image RNA-seq (paired-end 100 nucleotide reads) was performed on CM and CF polyA-selected RNA producing >160 million read pairs per sample with 85–90% mapping to the mouse genome ( Supplementary Table 1 ). Biological replicates generated highly reproducible results in neonatal CF and CM populations with high Pearson coefficients ( R ) for both gene expression ( R CM =0.98, R CF =0.99) and AS ( R CM =0.96, R CF =0.94). In addition, gene expression from CM and ventricle RNA-seq data highly correlated ( R =0.81) while CF-ventricle correlation was low ( R =0.33) ( Supplementary Fig. 2a–c ). These results are consistent with the fact that ~75% of the ventricular volume is formed by CM [7] . To evaluate CM and CF separation at all developmental stages, we used the fragments per kilobase per million mapped (FPKM) to estimate ‘CM enrichment’ (CME) and ‘CF enrichment’ (CFE) values defined as the ratios CM expression /CF expression and CF expression /CM expression , respectively [16] , [36] ( Fig. 3c ). This analysis provided several conclusions. First, while several CF-enriched transcripts showed constant ratios during development, CM-enriched transcripts showed a dramatic increase in CME values from PN1–3 to PN28. This reflects an active burst of CM maturation after birth compared with a less robust change during CF maturation (see below). Second, PN1–3 CME values were ≥10 for CM-enriched transcripts in PN1–3 and much higher for PN30 and adult indicating highly pure CM populations at all developmental stages. Third, the lower CFE values for some CF-enriched mRNAs at PN1–3 compared with PN30 and adult could reflect a low level of contamination as well as incomplete cell maturation. To evaluate possible contamination of the CF population with CM in PN1–3, we examined Nppa that is highly expressed in neonatal CM [28] . We found Nppa to be highly enriched in CM compared with CF populations and estimate contamination of CF preparations (PN1–3) with CM to be <2%. Reciprocal gene expression transitions between CM and CF RNA-seq revealed 3,064 downregulated genes in CM and 1,645 in CF from PN1–3 to adult. Upregulated genes numbered 1,981 in CM and 928 in CF. Interestingly, >82% of the differentially expressed genes in CM were not differentially expressed in CF ( Fig. 3d ). Postnatal gene expression transitions in CM and CF showed a reciprocal regulation of enriched functional categories such as mitochondrial metabolism, chemotaxis, cell adhesion and proliferation among others ( Fig. 3e , Supplementary Table 2 ). To validate reciprocal expression at the level of individual genes, we analysed expression of three previously published CM-specific genes involved in mitochondrial metabolism. RNA-seq data from CM and CF for Slc2a4 (solute carrier family 2, facilitated glucose), Cs (citrate synthase) and Pdk2 (pyruvate dehydrogenase kinase 2) transcripts showed postnatal upregulation for CM and downregulation for CF ( Fig. 3f ). The fold induction observed by RNA-seq in CM for these metabolic transcripts was comparable to quantitative PCR (qPCR) data previously reported in total mouse heart [28] . AS transitions in ventricles occur mainly before PN28 We next focused on AS transitions during postnatal heart development. AS assayed by either RNA-seq or RT–PCR was quantified as the PSI of the variable region and the change in splicing is ΔPSI [26] . To validate postnatal transitions detected by RNA-seq in ventricular RNA, we performed RT–PCR analysis of 36 events, 17 with ΔPSI≥20% predicted from RNA-seq, 8 with ΔPSI≤−20% and 11 with intermediate changes. A high Pearson correlation ( R =0.93) between ΔPSI values from RT–PCR and RNA-seq experiments demonstrated the accuracy of our RNA-seq data for both strongly and weakly regulated transitions ( Fig. 4a,b , Supplementary Fig. 3 and Supplementary Table 3 ). 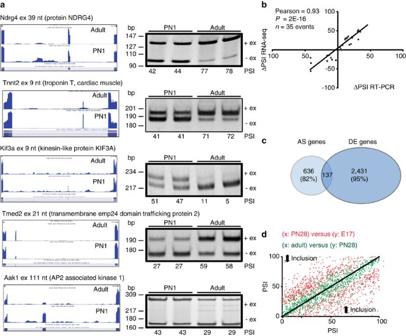Figure 4:Extensive postnatal AS transitions occur primarily without changes in gene expression. (a) RNA-seq data (UCSC browser) and RT–PCR assays (n=2 biological replicates) for AS events developmentally regulated (+ex: exon included; −ex: exon skipped). SeeSupplementary Fig. 3andSupplementary Table 3. (b) Correlation between RNA-seq and RT–PCR ΔPSI values.P, Student T distribution. (c) Genes undergoing postnatal AS transitions (|ΔPSI|≥20%) were intersected with differentially expressed (DE) genes in ventricles (E17-adult). (d) AS transitions (|ΔPSI|≥20%; E17-adult) were plotted comparing their change between E17–PN28 (red) and PN28-adult (green). Diagonal line: no difference between time points. Dots above/below the diagonal: increased/decreased inclusion. AS, alternative splicing; bp, base pairs; PSI, percent spliced in. Figure 4: Extensive postnatal AS transitions occur primarily without changes in gene expression . ( a ) RNA-seq data (UCSC browser) and RT–PCR assays ( n =2 biological replicates) for AS events developmentally regulated (+ex: exon included; −ex: exon skipped). See Supplementary Fig. 3 and Supplementary Table 3 . ( b ) Correlation between RNA-seq and RT–PCR ΔPSI values. P , Student T distribution. ( c ) Genes undergoing postnatal AS transitions (|ΔPSI|≥20%) were intersected with differentially expressed (DE) genes in ventricles (E17-adult). ( d ) AS transitions (|ΔPSI|≥20%; E17-adult) were plotted comparing their change between E17–PN28 (red) and PN28-adult (green). Diagonal line: no difference between time points. Dots above/below the diagonal: increased/decreased inclusion. AS, alternative splicing; bp, base pairs; PSI, percent spliced in. Full size image We identified 927 AS transitions during development (|ΔPSI|≥20%) in 773 genes, 82% occurring in genes for which transcript levels changed less than twofold ( Fig. 4c ). These results are consistent with previous evidence from a smaller set of AS transitions [3] . Therefore, a substantial impact of AS during development occurs through changes in protein isoform levels rather than total gene expression variations. As observed for gene expression transitions, the majority of the developmental AS changes occurred before PN28 ( Fig. 4d ). Temporal dynamics of AS transitions in CM and CF RNA-seq revealed that during postnatal development, more AS events changed in CM (809) than in CF (326) between neonatal and adult stages ( Fig. 5a ). Six transitions were validated in neonatal and adult CM and CF populations, showing high correlation ( R =0.84) between RT–PCR and RNA-seq ΔPSI values ( Supplementary Fig. 2d,e ). In both cell types, the majority of the events were cassette exons (82–83%) and the rest of them were alternative 3′-splice sites (6%), 5′-splice sites (7–9%) and intron retention (3–4%). There was a slight preference for inclusion of the variable region in both CM (65%) and CF (59%) during development ( Supplementary Fig. 2f,g ). 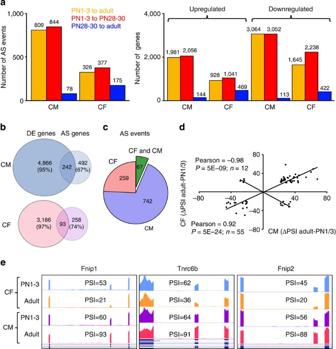Figure 5: Postnatal gene expression and AS transitions in CM and CF. (a) AS transitions (|ΔPSI|≥20%) and gene expression changes in CM and CF. (b) Genes developmentally regulated by splicing (|ΔPSI|≥20%) in CM and CF were intersected with differentially expressed (DE) genes (PN1–3 versus PN28–30). (c) Postnatal AS transitions (between PN1–3 and adult) specifically in CM, CF or both. (d) Analysis of the 67 events regulated in CF and CM.P, Student T distribution. (e) Three postnatal AS transitions occurring in opposite directions in CM and CF. AS, alternative splicing; PSI, percent spliced in. Figure 5: Postnatal gene expression and AS transitions in CM and CF. ( a ) AS transitions (|ΔPSI|≥20%) and gene expression changes in CM and CF. ( b ) Genes developmentally regulated by splicing (|ΔPSI|≥20%) in CM and CF were intersected with differentially expressed (DE) genes (PN1–3 versus PN28–30). ( c ) Postnatal AS transitions (between PN1–3 and adult) specifically in CM, CF or both. ( d ) Analysis of the 67 events regulated in CF and CM. P , Student T distribution. ( e ) Three postnatal AS transitions occurring in opposite directions in CM and CF. AS, alternative splicing; PSI, percent spliced in. Full size image Consistent with the AS analysis from ventricular RNA, >90% of postnatal transitions in CM occurred by PN30 (844 versus 78 after PN30). In CF, less than half of the postnatal transitions occurred before PN28 (377 versus 175 after PN28; Fig. 5a , left). These results suggest that AS primarily affects CM maturation during the first 4 weeks after birth while in CF splicing changes are distributed throughout postnatal life. Gene expression patterns showed a similar burst of expression before PN28–30 that was more pronounced in CM than in CF ( Fig. 5a , right). More than half of the genes undergoing postnatal AS transitions in either CM (67%) or CF (74%) did not change expression ≥2.0-fold and the majority of postnatal transitions were specific to either CM or CF populations ( Fig. 5b,c ). Only 67 events were developmentally regulated in both cell types, 82% of them (55 events) occurred in the same direction and 12 events showed opposite transitions in CF and CM with a strong negative correlation ( R =−0.98; Fig. 5d,e ). Taken together, these data confirmed that, as in ventricles, AS transitions occur primarily by PN28 in CM and are mainly cell-type specific. Postnatal regulation of vesicular trafficking genes by AS The AS transitions in ventricles (E17-adult) showed that vesicular trafficking, protein localization transport, endocytosis, membrane organization and invagination were the most represented categories ( P <5E−03, Fisher exact test) including the largest numbers of genes (10–27). Analysis of three time windows (E17–PN1, PN1–PN28 and PN28-adult) revealed that categories related to vesicular trafficking and membrane organization were enriched and highly significant before PN28. In contrast, categories related to transcription regulation and chromatin organization were predominant after PN28 ( Fig. 6a ). In general, GO analysis of AS and differentially expressed genes showed little overlap, further suggesting independence of AS and gene expression regulation ( Figs 2a,c , 3e and 6a,b ). 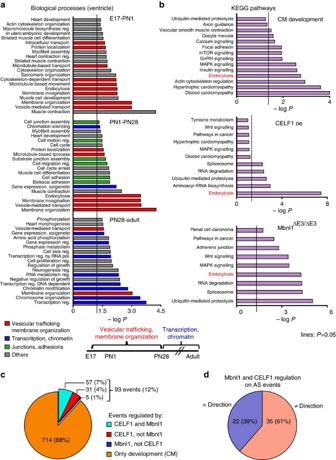Figure 6: Vesicular trafficking genes are regulated by AS during development. (a) GO analysis on AS genes (|ΔPSI|≥20%) in three time windows: E17–PN1, PN1–PN28 and PN28-adult (ventricles).P, Fisher exact test. (b) The Kyoto Encyclopedia of Genes and Genomes pathway analysis on AS genes detected by RNA-seq during wild-type CM development (|ΔPSI|≥20%) in adult CELF1-expressing hearts (CELF1 oe) and adultMbnl1ΔE3/ΔE3hearts (|ΔPSI|≥10%).P, Fisher exact test. (c) AS transitions (|ΔPSI|≥20%) during CM development (between PN1–3 and adult): regulation by Mbnl1 and/or CELF1. (d) The 57 events regulated by Mbnl1 and CELF1 were analysed in terms of antagonistic/non-antagonistic effects (Supplementary Table 4). AS, alternative splicing. Figure 6: Vesicular trafficking genes are regulated by AS during development. ( a ) GO analysis on AS genes (|ΔPSI|≥20%) in three time windows: E17–PN1, PN1–PN28 and PN28-adult (ventricles). P , Fisher exact test. ( b ) The Kyoto Encyclopedia of Genes and Genomes pathway analysis on AS genes detected by RNA-seq during wild-type CM development (|ΔPSI|≥20%) in adult CELF1-expressing hearts (CELF1 oe) and adult Mbnl1 ΔE3/ΔE3 hearts (|ΔPSI|≥10%). P , Fisher exact test. ( c ) AS transitions (|ΔPSI|≥20%) during CM development (between PN1–3 and adult): regulation by Mbnl1 and/or CELF1. ( d ) The 57 events regulated by Mbnl1 and CELF1 were analysed in terms of antagonistic/non-antagonistic effects ( Supplementary Table 4 ). AS, alternative splicing. Full size image Vesicular trafficking categories were also highly predominant during CM development ( Fig. 6b ) while transitions during CF development were enriched for other Kyoto Encyclopedia of Genes and Genomes pathways (adherens junction, P =1E−02; actin-cytoskeleton regulation, P =5E−02; ECM-receptor interaction, P =8E−02, Fisher exact test). Therefore, AS regulates different processes in each cell type. AS regulation of trafficking genes by Celf1 and Mbnl1 Celf1 and Mbnl1 have been shown to regulate AS during mouse heart development [3] , [37] , [38] . We used the RNA-seq data obtained from adult TRECUGBP1/MHC animals after 12, 24, 72 h or 7 days of doxycycline induction and MHC littermates (72 h on doxycycline) to identify CELF1-responsive AS transitions. Published RNA-seq data from hearts of Mbnl1 knockout mice ( Mbnl1 ΔE3/ΔE3 ) [39] allowed the identification of Mbnl1-sensitive events among postnatal AS transitions. From the 88 developmental transitions responsive to CELF1 re-expression in adults, 71 (81%) reverted to neonatal patterns. Of the 62 Mbnl1-sensitive transitions, 38 (61%) reverted to neonatal patterns in adult Mbnl1 ΔE3/ΔE3 animals. Overall, 93 postnatal AS transitions (12%) were regulated by CELF1 and/or Mbnl1 and more than half of them (57 events) were regulated by both (35 events antagonistically, 22 events in the same direction; Fig. 6c,d , Supplementary Table 4 ). Genes with postnatal AS transitions affected by CELF1 and/or Mbnl1 were enriched for vesicular trafficking, endocytosis and membrane organization-invagination processes ( Fig. 6b ). Reversion to neonatal splicing pattern in trafficking genes by CELF1 expression was confirmed by RT–PCR analysis of 17 events ( Fig. 7a–c , Supplementary Fig. 4 ). A high correlation was observed between RNA-seq and RT–PCR ΔPSI values and between developmental change (ΔPSI adult-PN1 ) and reversion after CELF1 expression (ΔPSI MHC-CELF1oe ) ( Fig. 7b,c ). The vesicular trafficking genes regulated by AS during development and responsive to CELF1 re-expression in adults are linked with each other after testing network connections using GeneMANIA software ( Fig. 7d ). 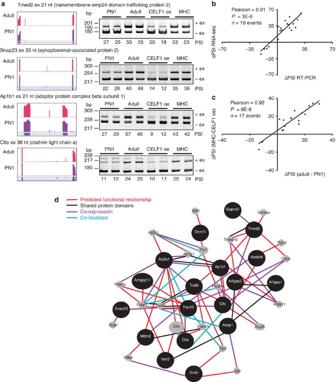Figure 7: Vesicular trafficking genes revert to neonatal splicing patterns after CELF1 re-expression in adult hearts. (a) RT–PCR (ventricles) of vesicular trafficking AS events during development and in CELF1-expressing hearts. Bar graphs: mean±s.e.m (n=2 biological replicates). (b) Correlation between RNA-seq and RT–PCR data in vesicular trafficking genes (PN1-adult).P, Student T distribution. (c) Correlation between developmental transitions in vesicular trafficking genes and reversion after CELF1 re-expression in adults (RT–PCR).P, Student T distribution. (d) Network of vesicular trafficking genes developmentally regulated by splicing and responsive to CELF1 (black circles). Grey circles: linking genes. CELF1 oe:TRECUGBP1/MHCanimals.MHC: control animals. bp, base pairs; PSI, percent spliced in. Figure 7: Vesicular trafficking genes revert to neonatal splicing patterns after CELF1 re-expression in adult hearts. ( a ) RT–PCR (ventricles) of vesicular trafficking AS events during development and in CELF1-expressing hearts. Bar graphs: mean±s.e.m ( n =2 biological replicates). ( b ) Correlation between RNA-seq and RT–PCR data in vesicular trafficking genes (PN1-adult). P , Student T distribution. ( c ) Correlation between developmental transitions in vesicular trafficking genes and reversion after CELF1 re-expression in adults (RT–PCR). P , Student T distribution. ( d ) Network of vesicular trafficking genes developmentally regulated by splicing and responsive to CELF1 (black circles). Grey circles: linking genes. CELF1 oe: TRECUGBP1/MHC animals. MHC : control animals. bp, base pairs; PSI, percent spliced in. Full size image We analysed the direct involvement of CELF1 in regulating AS during CM development by performing a motif analysis within the up- and downstream flanking introns (300 bp) of the exons regulated during development that responded to CELF1 re-expression in adults (88 events). GU-rich motifs were enriched ( P ≤1E−08, hypergeometric test) in downstream regions of AS exons ( Supplementary Fig. 5a ). Upstream flanking regions of AS exons were enriched in U- or C-rich motifs ( P =1E−14, hypergeometric test) when the variable regions were more skipped after CELF1 induction and GU-rich sequences ( P ≤1E−09, hypergeometric test) when the exons were more included in response to CELF1 ( Supplementary Fig. 5b ). iCLIP-seq data are available for Celf1 in C2C12 muscle cell differentiation [40] and were used for evidence of direct binding of Celf1 to the 71 transcripts regulated by AS during heart development that show a reversion to the neonatal pattern after CELF1 re-expression in adults. We evaluated the presence of iCLIP-tags within the up- and/or downstream 500 bp of the intron sequences flanking the AS exons and observed that 54% of them (38 out of 71) contain iCLIP-tags within these regions ( Supplementary Table 5 ; Fisher’s test: 1.7E−11 compared with whole gene exon iCLIP binding). When iCLIP-tags were evaluated for AS exons of vesicular trafficking genes, we found that 50% of them contain iCLIP-tags within 500 bp of their flanking regions; two examples are shown in Supplementary Fig. 5c . Taken together, these results support the hypothesis that vesicular trafficking is regulated at the splicing level during postnatal CM development and that CELF1 directly regulates a substantial fraction of these transitions. T-tubule and calcium release disruption by CELF1 induction Membrane organization and vesicular trafficking are particularly dynamic during postnatal CM development. The assembly of the excitation-contraction apparatus starts at birth and ends within 4 weeks involving T-tubule invagination from the sarcolemma, SR formation and vesicular trafficking of ion channels and adaptor proteins to specialized membrane regions [41] , [42] . We hypothesized that the splicing transitions regulated by Celf1 play a role in assembly and maintenance of these structures. To test this hypothesis, we determined the effect of CELF1 induction on adult T-tubule structure and function. CELF1 was re-expressed in adult mice for 4 days specifically in CM ( Fig. 8a ). CELF1-expressing animals showed altered electro- and echocardiograms exhibiting lower fractional shortening, ejection fraction and heart rate compared with MHC controls ( Fig. 8b , Supplementary Tables 6 and 7 ). The animals with higher exogenous CELF1 expression (#4) showed more affected cardiac parameters than the animal with lower exogenous CELF1 expression (#3). T-tubules were stained and imaged in living CM ( Fig. 8c ) and T-tubule structure was studied by three approaches. First, we delimited a rectangular region within the cell excluding nuclei and we performed the fast Fourier transform (FFT), an algorithm to convert a function of time/space into a frequency function and vice versa . With the FFT, we obtained the normalized T-tubule power by measuring the ratio between the pick power (first pick of the FFT) and the baseline power. Normalized T-tubule power after FFT measures the global regularity of the T-tubule network, and densities of transverse and longitudinal elements of T-tubules [41] , [43] (see Methods). CELF1-expressing CM showed lower T-tubule power than MHC controls ( Fig. 8d ). Second, we quantified the average T-tubule area within CM [28] . T-tubule area is defined as the percentage of the area containing T-tubule staining [28] (see Methods). While MHC mice showed 18±3% ( n =12 cells) of CM area as T-tubules, CELF1-expressing CM showed 9±1% ( n =16 cells; P =0.02, Student's t -test; Fig. 8e ). When analysed separately, CM from mice expressing higher CELF1 levels showed less T-tubule area compared with mice expressing lower CELF1 levels (mouse #3: 12±1%, mouse #4: 7±1%). Third, we devised an approach to estimate the proportion of individual cells with disorganized T-tubule structure (T-tubule irregularity; see Methods). Control CM showed lower T-tubule irregularity (10±2%; n =13 cells) than CELF1-expressing CM (36±5%; n =16 cells; P =4E−05, Student's t -test; Fig. 8f ). 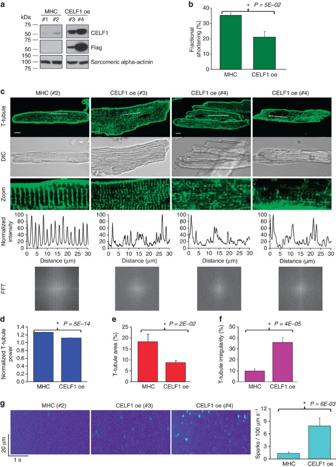Figure 8: T-tubule disorganization after CELF1 re-expression in adults. (a) Western blot analysis from adult hearts after CELF1 induction. (b) Fractional shortening was measured inMHC(n=6 animals) andTRECUGBP1/MHCmice (n=3 animals) that were given doxycycline (4 days). Results are expressed as the mean±s.e.m. (c) Confocal imaging of T-tubules on living CM fromMHC(#1–2;n=2 animals) and CELF1-expressing (#3–4,n=2 animals) mice. Scale bar, 10 μm. Third row: fluorescence plot over the white line on the first row. (d–g) T-tubule and calcium spark analysis: normalized T-tubule power (d) (n=13 cells for MHC animals,n=16 cells forTRCUGBP1/MHCanimals), T-tubule area (e) (n=12 cells forMHCanimals,n=16 cells forTRCUGBP1/MHCanimals), T-tubule irregularity (f) (n=13 cells forMHCanimals,n=16 cells forTRCUGBP1/MHCanimals), calcium spark frequency (g) (n=11 cells per genotype). *P≤0.05, Student'st-test. Results are expressed as the mean±s.e.m. CELF1 oe:TRECUGBP1/MHCanimals. MHC: controls. DIC, differential interference contrast microscopy; FFT, fast Fourier transform; T-tubules, transverse tubules. Figure 8: T-tubule disorganization after CELF1 re-expression in adults. ( a ) Western blot analysis from adult hearts after CELF1 induction. ( b ) Fractional shortening was measured in MHC ( n =6 animals) and TRECUGBP1/MHC mice ( n =3 animals) that were given doxycycline (4 days). Results are expressed as the mean±s.e.m. ( c ) Confocal imaging of T-tubules on living CM from MHC (#1–2; n =2 animals) and CELF1-expressing (#3–4, n =2 animals) mice. Scale bar, 10 μm. Third row: fluorescence plot over the white line on the first row. ( d – g ) T-tubule and calcium spark analysis: normalized T-tubule power ( d ) ( n =13 cells for MHC animals, n =16 cells for TRCUGBP1/MHC animals), T-tubule area ( e ) ( n =12 cells for MHC animals, n =16 cells for TRCUGBP1/MHC animals), T-tubule irregularity ( f ) ( n =13 cells for MHC animals, n =16 cells for TRCUGBP1/MHC animals), calcium spark frequency ( g ) ( n =11 cells per genotype). * P ≤0.05, Student's t -test. Results are expressed as the mean±s.e.m. CELF1 oe: TRECUGBP1/MHC animals. MHC: controls. DIC, differential interference contrast microscopy; FFT, fast Fourier transform; T-tubules, transverse tubules. Full size image Next, we addressed whether T-tubule disruption correlated with defective calcium release. Calcium spark frequency was higher in CELF1-expressing CM than in controls (7.9±1.9 versus 1.4±0.4 sparks (100 μm) −1 sec −1 ; n =11 cells each genotype; P =6E−03, Student's t -test; Fig. 8g ). Similar to T-tubule disruption, CELF1-expressing mouse #4 (sicker) presented more frequent calcium sparks than CM from mouse #3 (healthier; 10±3 versus 6±2 sparks (100 μm) −1 sec −1 ). Spontaneous calcium sparks are due to the opening rate of ryanodine receptors and frequency changes reflect alterations in ryanodine receptor itself, its association with other proteins, receptor cluster spatial organization, inter-cluster distance and/or calcium content in the SR [44] . Overall, T-tubule organization observed in CELF1-expressing CM resembles PN10–15 structure [41] , suggesting reversion to earlier developmental stages. We used RNA-seq to identify transcriptome dynamics from late embryonic to adult mouse heart development. While multiple studies have focused on specific genes or gene sets during heart development, this study presents a global analysis of postnatal gene expression and AS transitions in ventricles and freshly isolated CM and CF. The strong correlations of global postnatal changes between CM and ventricles flash frozen immediately after the euthanasia supports our contention that transcriptome transitions identified in isolated CM and CF are largely representative of those occurring in tissue. The similarity between ventricle and CM RNA-seq data is particularly striking, given that CM RNA was polyA selected and ventricular RNA was prepared by rRNA depletion. Overall, we revealed novel insight into strikingly different postnatal gene expression and AS transitions that occur in distinct but highly interacting cell populations within ventricles. The largest transitions between E17-adult occur before PN28, a period in which extensive physiological changes take place as the fetal heart adapts to birth and converts to adult function [1] , [2] . In CM, 90% of the gene expression and AS transitions occur before PN28 while in CF nearly 50% occur later. Gene expression and AS follow the same patterns in each cell type suggesting a general tendency for CM to set an adult pattern of gene output within the first 4 weeks after birth while CF undergo a more gradual transition. We hypothesize that this reflects the maturation required in CM in response to cell proliferation loss, cellular hypertrophy and rapidly increasing workload during the first 4 weeks after birth. By contrast, CF would not require as dramatic physiological maturation. Our data reveal a high level of specificity in CM and CF gene expression and a reciprocal expression changes in the two cell types. While genes involved in critical CM functions such as mitochondrial metabolism are developmentally upregulated, they are downregulated in CF. Similarly, focal adhesions and chemotaxis genes are upregulated during CF development but downregulated in CM. We examined potential mechanisms for post-transcriptional regulation of gene expression during development and identified a likely role for the 10-fold downregulation of Celf1 in the developmental upregulation of a subset of genes. While our previous analysis focused on the Celf1 role in a set of splicing transitions [3] , Celf1 has also been shown to destabilize mRNAs by binding to GU-rich motifs within 3′-UTRs [34] , [35] . We showed that 41% of the genes normally upregulated during development were downregulated on CELF1 induction and from those GU-rich motifs are enriched in 3′-UTRs of mitochondrial metabolism genes. Therefore, our results implicate Celf1 in coordinated upregulation of genes involved in the postnatal metabolic transition of CM. Consistent with our previous smaller-scale study [3] , the majority of AS transitions detected during postnatal heart development occurs without changes in total gene output, indicating that protein isoform switches are important regulatory components during postnatal development. Categories highly regulated by AS in heart, specifically in CM, are vesicular trafficking, endocytosis, membrane organization invagination. A link between trafficking and AS is novel, although several individual AS events in trafficking genes (for example, Snap25, Dab2 and Mdm2 ) have been reported [45] , [46] . In addition, categories relevant to trafficking were enriched among genes modulated by AS by CELF1 and Mbnl1, suggesting that these developmentally regulated RNA-binding proteins play a role in vesicle-mediated transport and membrane remodelling in CM. Membrane remodelling and endocytosis are crucial in eukaryotic cells for a variety of functions, some of which are cell-type specific [47] . Recently, it was reported that AS has an impact on endocytosis during brain development, suggesting that vesicular trafficking functions are coordinated by AS [21] . Our results are similar in heart and the impact of vesicular trafficking on cardiac functions is not known. Although many differences exist between the heart and brain, parallels between neuroscience and cardiac fields are growing, particularly with regard to ion channels and vesicular trafficking processes [48] . We hypothesize several non-exclusive scenarios for vesicular trafficking roles during postnatal heart development. First, AS regulation of vesicle-mediated transport could reflect changes in ligand/growth factor uptake during development. Second, after PN7, CM stop dividing and undergo cellular hypertrophy [14] , [15] . The most rapid increase in CM volume occurs between PN4 and PN20, after which CM volume increases only slightly [49] . Therefore, cells must maintain the appropriate internalization-recycling balance while membrane exposure to the extracellular environment is rapidly increasing. Third, vesicular trafficking regulation by AS could control the dynamics of ion channel production and localization. Ion channels are continuously formed, trafficked within vesicles for insertion and anchoring to specific subregions of the plasma membrane, and removed for degradation or recycling. Ion channel function is, therefore, dependent in part on surface density, which is tightly regulated by vesicular trafficking. The last scenario is supported by our analysis of T-tubule organization and function after CELF1 re-expression in adults. Maturation and assembly of SR and T-tubules in CM occur within the first 3–4 weeks after birth [41] producing the machinery for ECC. These maturation processes involve extensive cell architecture transitions, including membrane re-organization and vesicular-mediated protein transport. Membrane invagination and vesicular trafficking are regulated by AS during postnatal development and this may have an impact on CM functions such as ECC and uptake, distribution and recycling of key molecules (ion channels, growth factors and receptors). Importantly, both upregulation of CELF1 and loss of MBNL1 function are involved in the pathogenic mechanisms of myotonic dystrophy type 1 in which the best characterized molecular feature is expression of fetal AS splicing patterns [50] . The alterations in T-tubule structure and function we demonstrated strongly correlate with the finding that 80% of individuals with myotonic dystrophy type 1 exhibit cardiac arrhythmias [51] . Materials Cell culture reagents were obtained from GIBCO, Life Technologies. Liberase TH Research Grade and Collagenase/Dispase enzymes were from Roche Applied Science. Animals Ventricles, CM and CF were isolated from FvB wild-type mice. TRECUGBP1/Myh6-rtTA ( TRECUGBP1/MHC ) mice were used for human CELF1 overexpression in CM (tetracycline inducible) as described [3] , [33] . Bitransgenic and Myh6-rtTA ( MHC ) control adult animals were fed 2 g kg −1 doxycycline (BioServ) for 12, 24, 72 h and 7 days (RNA-seq), 8 days (RT–PCR) or 4 days (T-tubule/calcium experiments). We followed the NIH guidelines for use and care of laboratory animals approved by Baylor College of Medicine Institutional Animal Care and Use Committee. Ventricle heart isolation Animals were anaesthetized and after cervical dislocation (older than PN10) or decapitation (neonatal) hearts were removed. Blood and atria were removed; ventricles were frozen in liquid nitrogen or freshly used for CM and CF isolation. CF and CM isolation PN28 and adult CF isolation by pre-plating method. Minced ventricles were digested in DMEM containing 0.1 U ml −1 Collagenase, 0.8 U ml −1 Dispase and 0.1% EDTA-free Tripsin for 10 min at 37 °C (with stirring). After sedimentation the remaining tissue was similarly digested for 10 min. The suspension was centrifuged for 5 min at 3,000 g , cells were re-suspended in MEM-α supplemented with 10% fetal bovine serum and kept on ice. This procedure was repeated 3–4 times, cells were centrifuged for 5 min at 3,000 g , the pellet was re-suspended in MEM-α/20% fetal bovine serum and cells were seeded on cell culture dishes. Cells were plated for 2 h at 37 °C under 5% CO 2 . Adherent cells were washed 10 times with PBS and RNA was immediately extracted. Neonatal CF and CM isolation . The neonatal CM isolation kit (Cellutron Life Technology) was used with 20–35 ventricles accordingly to the manufacturer’s protocols. PN30 and adult CM isolation by Langendorff perfusion . The heart was removed with the lungs without touching the heart, rinsed in Ca 2+ free Tyrode’s solution (140 mM NaCl, 5.4 mM KCl, 1 mM MgCl 2 , 10 mM glucose, 5 mM HEPES pH 7.4) and cleaned from fat tissue. The heart was cannulated through the aorta and perfused on a Langendorff apparatus with Ca 2+ -free Tyrode’s solution for 3–5 min, and then with Ca 2+ -free Tyrode’s solution containing 20 μg ml −1 (0.104 Wünsch units ml −1 ) Liberase for ~15–25 min at 37 °C and then with KB solution (90 mM KCl, 30 mM K 2 HPO 4 , 5 mM MgSO 4 , 5 mM pyruvic acid, 5 mM β-hydroxybutyric acid, 5 mM creatinine, 20 mM taurine, 10 mM glucose, 0.5 mM EGTA, 5 mM HEPES pH 7.2) to wash out the enzyme. Atria were removed, the heart was minced in KB solution, cells were gently pipeted up and down (on ice) and filtered through Nylon mesh 210 μm open 155 μm thread, 24′ × 12′ mesh (Small Parts Inc). The sample was centrifuged for 5 min at 3,000 g and RNA was immediately extracted, or fresh CM were used for T-tubule experiments or immunofluorescences, or were frozen in liquid nitrogen for western blot assays. RNA extraction RNeasy fibrous tissue mini-kit (ventricles and CM) and RNeasy micro-kit (CF) were used (QIAGEN). RNA-seq analysis of CM and CF during development RNA-seq samples showed the following parameters: A 260nm / A 280nm ≥1.8, A 260nm / A 230nm ≥1.4, r28S:16S≥1.5 and RNA integrated number ≥8.6. Illumina TruSeq RNA sample preparation protocols were used for CM (PN1–2, PN1, PN30 and PN67) and CF (PN1–3, PN1–2, PN28 and PN60). In brief, a double-stranded DNA library was created using 1 μg total RNA. First, cDNA was created using the fragmented 3′-poly(A)-selected portion of total RNA and random primers. Libraries were generated from the cDNA by blunt ending the fragments, attaching an adenosine to the 3′-end and finally ligating unique adapters to the ends. The ligated products were amplified by PCR (15 cycles). Libraries were quantified using the NanoDrop spectrophotometer and fragment size assessed with the Agilent Bioanalyzer. A qPCR was performed on the libraries to determine the concentration of adapter-ligated fragments using a Bio-Rad iCycler iQ Real-Time PCR Detection System and a KAPA Library Quant Kit. Using the concentration from the Bio-Rad qPCR, 11 pM library was loaded onto a flow cell and amplified by bridge amplification using the Illumina cBot equipment. A paired-end 100 cycle run was used to sequence the flow cell on a HiSeq Sequencing System. RNA-seq Illumina TruSeq protocols were used for wild-type CM (PN1–2, PN1, PN30 and PN67) and CF (PN1–3, PN1–2, PN28 and PN60), and ventricles from TRECUGBP1/MHC or MHC animals ( n =3 animals each time point). For developmental ventricle analysis, RNA was rRNA depleted and libraries were prepared by Ribo-Zero Magnetic Gold and ScriptSeq-v2 RNA-seq library preparation kits (Epicentre Biotechnologies). In brief, total RNA (2 μg) from ventricles of E17, PN1, PN10, PN28 and PN90 (adult) animals was rRNA depleted using the Ribo-Zero Magnetic Gold Kit following the manufacturer’s protocols. The rRNA-reduced samples (~30 ng) were fragmented and primed with random hexamers containing a 5′-tagging sequence for RT priming. The 5′-tagged first-strand cDNA was then generated. During the second-strand cDNA generation, the RNA templates were removed leaving the 5′-tagged strand. Terminal-tagging oligos were annealed to the 5′-tagged strand and terminal-tagging oligos were blocked at the 3′-end preventing the synthesis of a secondary strand. Resulting cDNA strand was single stranded and tagged at both ends. The di-tagged cDNA was purified using Agencourt AMPure XP system (Beckman Coulter). Single-stranded cDNA generated for each sample was used for library construction. Using PCR amplification (10 cycles), the second cDNA strand was generated and the Illumina adapter sequences were added simultaneously to the single-stranded di-tagged cDNA fragments. Illumina sequencing libraries were purified using Agencourt AMPure XP system. Libraries were validated on an Agilent Bioanalyzer High Sensitivity DNA chip checking the purity of the sample and the size of the insert. Libraries were within 150–2000, bp on the electropherogram. A second round of purification using Agencourt AMPure XP system was required for removal of primer-dimer and adapter-dimer contamination. Libraries were quantified using KAPA SYBR Fast qPCR kit from KAPA Biosystem. Libraries were diluted to 2 nM (based on cT values), alkali denatured for 5 min, diluted to a final concentration of 11 pM and dispensed into thin-walled PCR tubes to be loaded into the Illumina cBot. Clusters were generated on the flow cell by PCR with the Illumina cluster generation kit. The flow cell containing clustered libraries were loaded on the Illumina HiSeq instrument along with the kitted sequencing reagents for a paired-end (PE) 100 bp run. During each sequencing cycle, a dye-terminated nucleotide was incorporated into the single-stranded DNA strand and fluorescence was monitored. Fluorescent dye was cleaved to allow next nucleotide incorporation. CASAVA software converted the fluorescence measurements into sequence files. Computational processing of developmental RNA-seq data RNA-seq alignment . Paired-end RNA-seq reads were aligned to the mouse genome (mm9) using TopHat 2.0.5 (ref. 52 ). Differentially expressed gene analysis and FPKM . RSEM [53] was used to count the number of fragments mapped into Ensembl gene models, followed by edgeR [54] to call differentially expressed genes with false discovery rate less than 0.01. The gene expression was quantified by FPKM [55] . Differential AS events . On the basis of the Ensembl 65 gene model, SpliceTrap [56] was employed to identify differential exon skipping, intron retention events, alternative 5′- or 3′-splice site. AS was quantified by the percentage of mRNAs that contain an alternative region as PSI value. The events with PSI changes between two conditions |ΔPSI|≥20% were called differential splicing events. Computational processing of the CELF1 RNA-seq data Estimation of gene and isoform expression levels was performed in a manner similar to previously described [39] . In brief, reads were mapped to the mouse genome (mm9) and a database of splice junctions using the Bowtie tool [57] . Gene expression . Gene expression was measured as following: (i) the number of reads mapping to constitutive exons for each gene was measured and (ii) that measurement was divided by the number of kilobases of constitutive exon model per million uniquely mapped reads. AS events . Isoform levels and Bayes factors were measured by MISO [58] (single end mode). Bioinformatic analysis of 3′-UTRs The Database for Annotation, Visualization and Integrated Discovery v6.7 (refs 59 , 60 ) was used for GO analysis considering P ≤0.05 significant. miRNA prediction analysis was performed using TargetScan ( http://www.targetscan.org/ ) and motif analysis with CLIPZ (SIB) and MEME version 4.9.0 (ref. 61 ) (motif>6–18 bp) softwares. The E -value (MEME) is the enrichment of a motif based on its log likelihood ratio, width, sites, background frequencies and the training set size. The P value of a site is computed from the match score of the site with the position-specific scoring matrix for the motif. The P value gives the probability of a random string (generated from the background letter frequencies) having the same match score or higher. Gene network of AS genes involved in vesicular traffic, developmentally regulated and sensitive to CELF1 induction was performed using GeneMANIA [62] . Bioinformatic analysis of AS events The analysis involved the 88 developmental transitions responsive to CELF1 re-expression in adults. The 300 nucleotide upstream and downstream of the alternative spliced exons were used for de novo motif analysis, excluding the last 30 nucleotides of the upstream intron and first 9 nucleotides of the downstream intron of the alternative exons that contain the conserved 5′- and 3′-splice sites, respectively. Then motif analysis tool HOMER (v4.3) [63] was employed for RNA motif analysis with the background sequences generated by the first-order Markov model the parameters of which were estimated based on hg19. Celf1 HITS-Clip data analysis C2C12 Celf1 HITS-CLIP data were downloaded from the European Nucleotide Archive (accession code ERP000789) [64] . As described by authors [64] , the 4-bp tags were trimmed and sequences composed primarily of Illumina adapter were removed. The pre-processed reads were mapped to the mouse genome (mm9) using the alignment tool Bowtie [57] with allowed two mismatch. Finally, reads with identical 5′ starts were further collapsed into a single read to avoid potential PCR duplicates’ effects and only uniquely mapped reads were kept as final Celf1-binding tags. AS validations by RT–PCR RT–PCR was performed (High Capacity cDNA RT Kit, Applied Biosystems; and GoTaq DNA Polymerase, Promega) in biological duplicates and products were analysed by 6% PAGE. PCR reactions involved the following steps: (i) 95 °C for 3 min, (ii) 20–27 cycles of 95 °C for 30 s, 58 °C for 30 s and 72 °C for 30 s, (iii) 72 °C for 7 min and (iv) 25 °C for 5 min. RNA-seq data were used to design primers annealing in the constitutive flanking exons of the AS region. Sequences of the primers (SIGMA) used for validation in ventricles are shown in Supplementary Table 8 . Sequences of the primers (SIGMA) used for validation of AS events on vesicular trafficking-related genes are shown in Supplementary Table 9 . Densitometry measurements were performed using Kodak Gel logic 2200 and Molecular Imaging Software. PSI [26] was calculated by densitometry following equation (1). Analysis of CM and CF markers by RT–PCR RT–PCR assays were performed using the following primers (SIGMA): vimentin-F (5′-TGAAGGAAGAGATGGCTCGT-3′), vimentin-R (5′-TTGAGTGGGTGTCAACCAGA-3′), Ddr2-F (5′-CAAGATCATGTCTCGGCTCA-3′), Ddr2-R (5′-GCCCTGGATCCGGTAGTAAT-3′), Nkx2.5-F (5′-AAGCAACAGCGGTACCTGTC-3′), Nkx2.5-R (5′-GGGTAGGCGTTGTAGCCATA-3′), Tnnt2-F (5′-CGGAAGAGTGGGAAGAGACA-3′), Tnnt2-R (5′-TTCCCACGAGTTTTGGAGAC-3′), mGadph-F (5′-CGTCCCGTAGACAAAATGGT-3′) and mGadph-R (5′-TTGATGGCAACAATCTCCAC-3′). PCR reactions involved the following steps: (i) 95 °C for 75 s, (ii) 20–27 cycles of 95 °C for 45 s, 57 °C for 45 s and 72 °C for 1 min, (iii) 72 °C for 10 min and (iv) 25 °C for 5 min. PCR products were analysed by 6% PAGE. Immunofluorescence After adult CM and CF isolation, cells were seeded onto coverslips overnight (CM) or for 70 h (CF). Coverslips were pre-coated with 20 μg ml −1 laminin for 1 h at 37 °C for CM. Cells were fixed in 3.7% paraformaldehyde on ice for 20 min, blocked with PBS/0.3% TritonX-100/1% BSA for 1 h at 37 °C and incubated overnight at 4 °C with primary antibodies (rabbit monoclonal anti-vimentin (D21H3; Cell Signaling, #5741; 1:100) or mouse monoclonal (clone BM-75.2) anti-alpha-actinin (SIGMA, #A5044; 1:50). After washes, samples were incubated with secondary antibodies conjugated with Alexa-fluor-488 (Invitrogen; 1:500) for 1 h at 37 °C, washed, stained with 2 μM 4',6-diamidino-2-phenylindole (DAPI) for 5 min and mounted (Slow Fade Gold Antifade Reagent, Invitrogen). Confocal microscopy was performed with a Nikon A1-Rs inverted laser scanning microscope with a × 40 Plan-Fluor/1.3 numerical aperture oil-immersion objective. Excitation: argon multiline laser at 488 nm (Alexa-fluor-488) or a 404-nm diode at 38 mW (DAPI). Emission filters: band-pass 525/50 nm (Alexa-fluor-488), band-pass 450/50 nm (DAPI). Confocal images were processed with ImageJ. Background was subtracted and a median filter was applied (radius=1 pixel) for presentation. T-tubules analysis Isolated CM (adult TRECUGBP1/MHC or MHC doxycycline fed, n =2 animals each) were stained with 10 μM Di-8-ANEPPS (Invitrogen, #D3167) in KB solution for 15 min, washed and imaged by confocal microscopy (Zeiss LSM-510 microscope, × 40 oil-immersion objective). Excitation: argon multiline laser, 488 nm. Emission filter: long-pass 505 nm. Quantifications were performed using ImageJ: 1) a region of interest was selected covering longitudinally the CM avoiding the nuclei, FFT was obtained, power spectrum was computed and normalized (normalized T-tubule power) [41] ; 2) a threshold (MaxEntropy) was applied (ImageJ), cell interior was manually delimitated (excluding plasma membrane), areas with green signal were summed within the threshold and normalized to the total area (T-tubule area); 3) CM from MHC animals showed four to six T-tubules (10 μm) −1 (ImageJ); therefore, regions with four to six T-tubules (10 μm) −1 were considered ‘regular-regions’ otherwise ‘irregular-regions’. Three lines were drawn along each CM, plots were obtained, normalized to its maximum, a cutoff (15 units above the baseline) was determined and each line was analysed by the number of picks (T-tubules) above the cutoff (between 0 and 10, 5 and 15, 10 and 20, 15 and 25 μm and so on) computing the ‘regular-regions’ and the ‘irregular-regions’ (in μm). For each CM, the total length of the three lines and the total ‘irregular-regions’ were summed and T-tubule irregularity was calculated. Calcium sparks analysis The same samples were incubated with 3.5 μM fluo-4-acetoxymethyl ester (Invitrogen, #F14201) in Tyrode’s solution (1.8 mM Ca 2+ ; 1 h, room temperature), washed (15 min) and transferred to a chamber containing parallel platinum electrodes. Fluorescence images were recorded after pacing (10 V, 0.5 ms) from CM showing clear striation and normal contractility. Sparks were analysed using SparkMaster plugin (ImageJ). Western blots After perfusion, a portion of the ventricles from TRECUGBP1/MHC or MHC control animals were lysed in HEPES-sucrose buffer (10 mM HEPES pH 7.4, 0.32 M sucrose, 1 mM EDTA and proteases inhibitors) using Bullet blender (Next Advance) equipment and SDS was added (final concentration: 1% SDS). Samples were sonicated (3 min at 75 V: 30 s on and 30 s off) and centrifuged for 10 min at 14,000 r.p.m. at 4 °C. Supernatants were transferred to new tubes and protein concentration was estimated with Pierce BCA protein assay kit (Thermo Scientific). Samples were diluted in loading buffer (100 mM Tris–HCl pH 6.8, 4% SDS, 0.2% bromophenol blue, 20% glycerol, 200 mM β-mercaptoethanol), boiled for 5 min and total proteins (40 μg) were assayed by 10% SDS–PAGE. After transfer, membranes were blocked in 5% non-fat-dried milk/0.1% Tween-TBS buffer for 1 h, washed and incubated overnight at 4 °C with primary antibodies diluted in 5% milk/Tween-TBS buffer: mouse monoclonal anti-CUG-BP1, clone 3B1 (Milipore, #05-621; 1:1,000), rabbit polyclonal anti-sarcomeric alpha-actinin (Abcam, #ab72592; 1:2,000). The following day, membranes were incubated with secondary antibodies (1:5,000) for 1 h at room temperature: peroxidase-conjugated goat anti-mouse IgG light chain-specific (Jackson Immunoresearch, #115-035-174), goat anti-rabbit IgG horseradish peroxidase conjugated (Invitrogen, # 621234). Flag-tag was detected by monoclonal anti-FLAG M2 peroxidase (Sigma, #A8592; 1:1,000; 1 h at room temperature). Super Signal West Pico Chemiluminescent Substrate kit (Thermo Scientific) was used for developing. ECG and echocardiogram recording Echocardiograms were performed using a Vevo 770 Ultrasound equipment with a 707B probe for the cardiac analysis. The animals were sedated with 2% isoflurane for imaging. The m-mode images were analysed for data acquisition using the Vevo analysis package. The electrocardiograms (ECGs) were recorded using a Mouse Monitor made by Indus Instruments. Mice were lightly anaesthetized using 1.5% isoflurane and the paws were taped to the ECG leads. ECGs were recorded for leads I, II and III for each animal and analysed. Both ECGs and ultrasounds were performed in the Mouse Phenotyping Core at the Baylor College of Medicine. Statistic Results were expressed as the mean±s.e.m, P values were estimated using Student’s t -test (two tailed) and P ≤0.05 was considered significant. Accession codes: RNA-Seq data have been deposited at NCBI Gene Expression Omnibus under accession code GSE49906 (developmental series: ventricles, cardiomyocytes and cardiac fibroblasts) and GSE56185 (CELF1 data). How to cite this article: Giudice, J. et al. Alternative splicing regulates vesicular trafficking genes in cardiomyocytes during postnatal heart development. Nat. Commun. 5:3603 doi: 10.1038/ncomms4603 (2014).